Ultraviolet-B-mediated induction of protein–protein interactions in mammalian cells Light-sensitive proteins are useful tools to control protein localization, activation and gene expression, but are currently limited to excitation with red or blue light. Here we report a novel optogenetic system based on the ultraviolet-B-dependent interaction of the Arabidopsis ultraviolet-B photoreceptor UVR8 with COP1 that can be performed in visible light background. We use this system to induce nuclear accumulation of cytoplasmic green fluorescent protein fused to UVR8 in cells expressing nuclear COP1, and to recruit a nucleoplasmic red fluorescent protein fused to COP1 to chromatin in cells expressing UVR8-H2B. We also show that ultraviolet-B-dependent interactions between DNA-binding and transcription activation domains result in a linear induction of gene expression. The UVR8–COP1 interactions in mammalian cells can be induced using subsecond pulses of ultraviolet-B light and last several hours. As UVR8 photoperception is based on intrinsic tryptophan residues, these interactions do not depend on the addition of an exogenous chromophore. In optogenetics, proteins are engineered to contain a photoreceptor that triggers functionality when struck by a photon of a specific wavelength. Optogenetics has been mainly applied in the neurosciences, where stimulation of microbial opsins by light polarizes the membrane, offering temporally precise activation of defined neurons [1] . In the past years, the interest in optogenetics has expanded to other fields, with both red and blue light-sensitive proteins having been engineered to control protein localization, pathway activation and gene expression [2] , [3] , [4] , [5] , [6] . Yet, for versatility in experimental design, there is a need for development of multiple optogenetic systems, especially systems that do not require addition of exogenous chromophores and that respond to different wavelengths of light. In Arabidopsis thaliana , ultraviolet-B (280–315 nm) light induces an interaction of the photoreceptor UVR8 with its partner COP1 ( [7] , [8] ). Biochemical and structural data indicate that UVR8 contains a seven bladed β-propeller type domain that in the absence of ultraviolet-B forms a homodimer [7] , [9] , [10] . The dimer interface is rich in tryptophan (Trp) residues, several of which are physically close to each other. When excited by ultraviolet-B, the Trp aromatic residues, particularly Trp285, function as a chromophore triggering monomerization of UVR8 ( [7] , [9] , [10] ). Mutant versions of UVR8 with Trp285 to phenylalanine (UVR8 W285F ) or alanine (UVR8 W285A ) substitutions do not respond to ultraviolet-B and are in vivo constitutively dimeric and monomeric, respectively [7] . Upon monomerization, UVR8 interacts with the E3 ubiquitin ligase COP1 and the two proteins accumulate in the nucleus, where they regulate expression of genes that provide protection from ultraviolet-B ( [8] , [11] , [12] ). COP1 contains three domains that are important for its function: an N-terminal RING domain, a coiled-coil domain and a seven WD-40 repeat domain at its C-terminus [13] . The C-terminal 340 amino acids of COP1 (COP1 C340 ), corresponding to the WD-40 domain, are sufficient to interact with UVR8 in yeast [7] . Here, we describe a novel optogenetic system that utilizes the UVR8 and COP1 interacting modules to induce ultraviolet-B-dependent protein–protein interactions. This new system does not require an exogenous chromophore and utilizes a wavelength that does not interfere with the commonly used fluorescent reporter proteins. Ultraviolet-B induced protein translocation To setup a novel optogenetic system, we first examined whether UVR8 and COP1 C340 interact in a ultraviolet-B-dependent manner in mammalian cells. We fused UVR8 to green fluorescent protein (GFP) and COP1 C340 to a monomeric Cherry (mCh) fluorescent protein bearing also a nuclear localization signal (NLS) ( Fig. 1a , Supplementary Fig. S1 ). We then monitored the localization of GFP-UVR8 and mCh-NLS-COP1 C340 in U2OS cells by time-lapse microscopy. Before ultraviolet-B illumination, GFP-UVR8 localized mostly in the cytoplasm, whereas mCh-NLS-COP1 C340 was nuclear. After illumination with ultraviolet-B, GFP-UVR8 gradually concentrated in the nucleus over the course of an hour ( Fig. 1b ). In contrast, under the same conditions, ultraviolet-B light did not induce nuclear retention of the GFP-UVR8 W285F mutant, whereas GFP-UVR8 W285A was constitutively nuclear due to constitutive interaction with mCh-NLS-COP1 C340 ( Fig. 1c ). In cells that did not express mCh-NLS-COP1 C340 , ultraviolet-B did not induce nuclear localization of GFP-UVR8 and GFP-UVR8 W285A was constitutively cytoplasmic ( Supplementary Fig. S2 ). 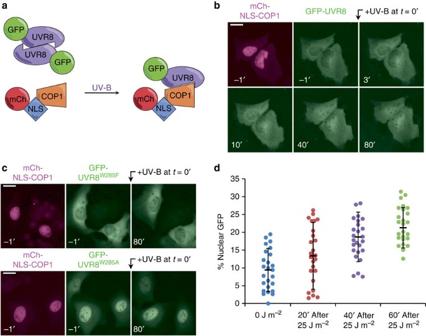Figure 1: Ultraviolet-B-dependent nuclear retention of GFP-UVR8. (a) Schematic representation of the ultraviolet-B-induced interaction of GFP-UVR8 with mCh-NLS-COP1C340. As a homodimer, GFP-UVR8 does not interact with mCh-NLS-COP1C340. After exposure to ultraviolet-B, the GFP-UVR8 dimer dissociates into monomers, each of which can interact with mCh-NLS-COP1C340. (b) Localization of GFP-UVR8 and mCh-NLS-COP1C340in U2OS cells before and after exposure to ultraviolet-B (25 J m−2). Timepoints in minutes, relative to the ultraviolet-B pulse, are indicated. Scale bar, 20 μm. (c) U2OS cells expressing GFP-UVR8W285For GFP-UVR8W285Aand mCh-NLS-COP1C340before and after a ultraviolet-B pulse (25 J m−2). Timepoints in minutes, relative to the ultraviolet-B pulse are indicated. Scale bar, 20 μm. (d) Fraction of nuclear GFP-UVR8 determined from analysis of live cell images before and after exposure to ultraviolet-B light. For each condition, 25 cells were analysed; circles indicate the values for each cell and lines show the means ± 1 s.d. of the mean. Figure 1: Ultraviolet-B-dependent nuclear retention of GFP-UVR8. ( a ) Schematic representation of the ultraviolet-B-induced interaction of GFP-UVR8 with mCh-NLS-COP1 C340 . As a homodimer, GFP-UVR8 does not interact with mCh-NLS-COP1 C340 . After exposure to ultraviolet-B, the GFP-UVR8 dimer dissociates into monomers, each of which can interact with mCh-NLS-COP1 C340 . ( b ) Localization of GFP-UVR8 and mCh-NLS-COP1 C340 in U2OS cells before and after exposure to ultraviolet-B (25 J m −2 ). Timepoints in minutes, relative to the ultraviolet-B pulse, are indicated. Scale bar, 20 μm. ( c ) U2OS cells expressing GFP-UVR8 W285F or GFP-UVR8 W285A and mCh-NLS-COP1 C340 before and after a ultraviolet-B pulse (25 J m −2 ). Timepoints in minutes, relative to the ultraviolet-B pulse are indicated. Scale bar, 20 μm. ( d ) Fraction of nuclear GFP-UVR8 determined from analysis of live cell images before and after exposure to ultraviolet-B light. For each condition, 25 cells were analysed; circles indicate the values for each cell and lines show the means ± 1 s.d. of the mean. Full size image To quantitate the ultraviolet-B-induced nuclear accumulation of GFP-UVR8 in cells expressing mCh-NLS-COP1 C340 , images of live cells were acquired at various times after exposure to a pulse of ultraviolet-B light and used to calculate the nuclear fraction of GFP-UVR8. The fraction of nuclear GFP-UVR8 increased over a 60-min time period after illumination with ultraviolet-B ( Fig. 1d ). As ultraviolet-B light induces an almost immediate UVR8 monomerization followed by interaction with COP1 ( [7] ), we speculate that the slow kinetics reflects inefficient transport of GFP-UVR8 from the cytoplasm to the nucleus, where it can be retained by mCh-NLS-COP1 C340 . As a second system to monitor ultraviolet-B-induced protein–protein interactions, we fused UVR8 to histone H2B and examined whether ultraviolet-B could be used to target nucleoplasmic COP1 C340 -fusion proteins to chromatin. Our initial UVR8 construct contained a single UVR8 moiety fused to H2B-GFP ( Supplementary Fig. S1 ). However, when we coexpressed H2B-GFP-UVR8 and mCh-NLS-COP1 C340 we observed constitutive interaction of the two proteins, independently of ultraviolet-B. We also observed constitutive interactions when mCh-NLS-COP C340 was coexpressed with H2B-GFP-UVR8 W285A and, even, with H2B-GFP-UVR8 W285F ( Supplementary Fig. S3 ). We speculated that the inter-nucleosome distance was too large to support dimerization of H2B-GFP-UVR8 molecules in the absence of ultraviolet-B. Thus, to allow the formation of UVR8 dimers, we fused H2B-GFP to two UVR8 moieties that were joined together by a 22-amino acid long flexible linker ( Fig. 2a , Supplementary Fig. S1 ). This fusion protein, referred to as H2B-GFP-UVR8(2x), did not recruit mCh-NLS-COP1 C340 to chromatin in the absence of ultraviolet-B. However, after a ultraviolet-B pulse, mCh-NLS-COP1 C340 localized to chromatin, indicating an interaction with H2B-GFP-UVR8(2x) ( Fig. 2b ). mCh-NLS-COP1 C340 remained bound to chromatin for at least 4 h after exposure to ultraviolet-B ( Supplementary Fig. S4a ). A mutant H2B-GFP-UVR8 W285F (2x) protein did not interact with mCh-NLS-COP1 C340 even after exposure to ultraviolet-B ( Fig. 2c ), while the H2B-GFP-UVR8 W285A (2x) mutant interacted constitutively with NLS-mCh-COP1 C340 ( Fig. 2d ). Similar results were obtained when, in place of a histone H2B moiety fused to the N-terminus of UVR8, a histone H3 moiety was attached to the UVR8 C-terminus ( Supplementary Figs S1,S4b ). 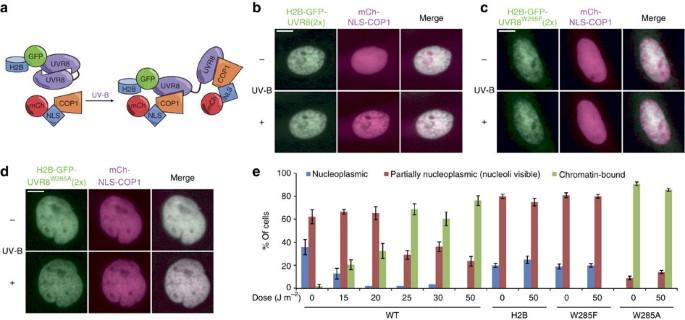Figure 2: Ultraviolet-B-dependent recruitment of mCh-NLS-COP1C340to chromatin. (a) Schematic representation of the ultraviolet-B-induced interaction of H2B-GFP-UVR8(2x) with mCh-NLS-COP1C340. In the absence of ultraviolet-B, the two UVR8 domains of H2B-GFP-UVR8(2x) interact with each other. After exposure to ultraviolet-B, this interaction is disrupted, allowing interaction with two mCh-NLS-COP1C340molecules. (b) Localization of H2B-GFP-UVR8(2x) and mCh-NLS-COP1C340before (−) and after (+) exposure to ultraviolet-B in U2OS cells. In this panel and in panelsc,dscale bar, 10 μm. (c) U2OS cells expressing mCh-NLS-COP1C340and H2B-GFP-UVR8W285F(2x) before (−) and after (+) ultraviolet-B illumination. (d) U2OS cells expressing mCh-NLS-COP1C340and H2B-GFP-UVR8W285A(2x) before (−) and after (+) ultraviolet-B illumination. (e) Quantification of localization patterns of mCh-NLS-COP1C340in U2OS cells co-expressing wild-type H2B-GFP-UVR8(2x) (WT), H2B-GFP (H2B) or the indicated H2B-GFP-UVR8(2x) mutants (W285A and W285F) before and after exposure to the indicated dose of ultraviolet-B. The bars indicate the means ± 1 s.e. obtained from five independent experiments. Figure 2: Ultraviolet-B-dependent recruitment of mCh-NLS-COP1 C340 to chromatin. ( a ) Schematic representation of the ultraviolet-B-induced interaction of H2B-GFP-UVR8(2x) with mCh-NLS-COP1 C340 . In the absence of ultraviolet-B, the two UVR8 domains of H2B-GFP-UVR8(2x) interact with each other. After exposure to ultraviolet-B, this interaction is disrupted, allowing interaction with two mCh-NLS-COP1 C340 molecules. ( b ) Localization of H2B-GFP-UVR8(2x) and mCh-NLS-COP1 C340 before (−) and after (+) exposure to ultraviolet-B in U2OS cells. In this panel and in panels c , d scale bar, 10 μm. ( c ) U2OS cells expressing mCh-NLS-COP1 C340 and H2B-GFP-UVR8 W285F (2x) before (−) and after (+) ultraviolet-B illumination. ( d ) U2OS cells expressing mCh-NLS-COP1 C340 and H2B-GFP-UVR8 W285A (2x) before (−) and after (+) ultraviolet-B illumination. ( e ) Quantification of localization patterns of mCh-NLS-COP1 C340 in U2OS cells co-expressing wild-type H2B-GFP-UVR8(2x) (WT), H2B-GFP (H2B) or the indicated H2B-GFP-UVR8(2x) mutants (W285A and W285F) before and after exposure to the indicated dose of ultraviolet-B. The bars indicate the means ± 1 s.e. obtained from five independent experiments. Full size image To quantify the dose required to induce recruitment of NLS-mCh-COP1 C340 to chromatin, we examined over 100 cells, per condition, after administering various doses of ultraviolet-B. We identified three mCh-NLS-COP1 C340 localization patterns: nucleoplasmic (where mCherry is distributed equally throughout the nucleus); partially nucleoplasmic (where mCherry is principally nucleoplasmic, but partially excluded from the nucleoli) and chromatin-bound (where mCherry colocalized with GFP-labelled H2B) ( Supplementary Fig. S5 ). As the dose of ultraviolet-B increased, the percentage of cells exhibiting the chromatin-bound pattern increased, with a plateau being reached at around 25 J m −2 ( Fig. 2e ). In the cells, that were not exposed to ultraviolet-B or that expressed H2B-GFP or H2B-GFP-UVR8 W285F (2x), mCh-NLS-COP1 was nucleoplasmic; whereas, in cells expressing the H2B-GFP-UVR8 W285A (2x) mutant, mCh-NLS-COP1 was constitutively chromatin-bound ( Fig. 2e ). These results suggest a tight regulation of the UVR8–COP1 interaction by ultraviolet-B light and by amino-acid substitutions affecting UVR8 dimerization in the nuclei of mammalian cells. Activation of transcription induced by ultraviolet-B light To establish whether protein–protein interactions relying on ultraviolet-B-dependent UVR8–COP1 heterodimerization could be used to regulate biological activities, we fused the transcription activation domain of NF-κB to UVR8 and the GAL4 DNA-binding domain to COP1 C340 ( Fig. 3a , Supplementary Fig. S1 ). We then expressed these proteins together with luciferase reporter plasmids in U2OS cells and measured luciferase activity as a function of exposure to ultraviolet-B light. In the absence of ultraviolet-B, luciferase activity was almost undetectable. In contrast, ultraviolet-B illumination induced a dose-dependent increase in luciferase activity that reached a plateau at a dose of about 25 J m −2 ( Fig. 3b ). Similar dose dependency, ultraviolet-B specificity and tightness of regulation were observed in a ultraviolet-B light-switchable gene expression system based on a two-hybrid interaction in yeast ( Supplementary Fig. S6 ). 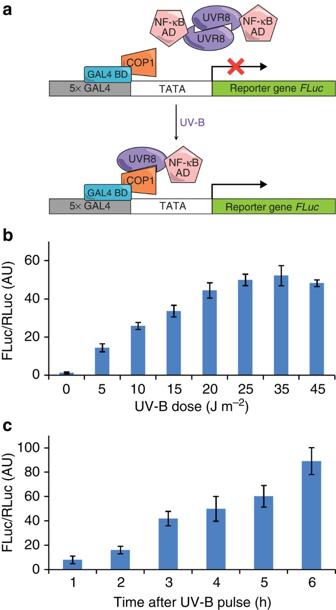Figure 3: Ultraviolet-B-dependent induction of transcriptional activity. (a) Schematic representation of the ultraviolet-B-induced interaction of the NF-κB activation domain (AD)-UVR8 fusion protein with the GAL4 DNA-binding domain (BD)-COP1C340-fusion protein and subsequent activation of transcription of a firefly luciferase (FLuc) gene driven by five GAL4 response elements. (b,c) Ratio of FLuc toRenillaluciferase (RLuc) activity as a function of exposure to ultraviolet-B. Expression of RLuc is driven by a constitutive promoter. Inb, luciferase activity was determined 4 h after exposure to ultraviolet-B. Inc, luciferase activity was determined after exposure to a ultraviolet-B dose of 25 J m−2. The bars indicate the means ±1 s.e. obtained from four independent experiments. Figure 3: Ultraviolet-B-dependent induction of transcriptional activity. ( a ) Schematic representation of the ultraviolet-B-induced interaction of the NF-κB activation domain (AD)-UVR8 fusion protein with the GAL4 DNA-binding domain (BD)-COP1 C340 -fusion protein and subsequent activation of transcription of a firefly luciferase ( FLuc ) gene driven by five GAL4 response elements. ( b , c ) Ratio of FLuc to Renilla luciferase (RLuc) activity as a function of exposure to ultraviolet-B. Expression of RLuc is driven by a constitutive promoter. In b , luciferase activity was determined 4 h after exposure to ultraviolet-B. In c , luciferase activity was determined after exposure to a ultraviolet-B dose of 25 J m −2 . The bars indicate the means ±1 s.e. obtained from four independent experiments. Full size image Temporal and spatial control of protein–protein interactions In all the experiments described so far, the cells were exposed to ultraviolet-B light using a transilluminator. This means that the cells could not be observed under the microscope at the time of exposure to ultraviolet-B and that, at least, a minute elapsed while transferring the cells from the transilluminator to the microscope. To optimize the method, we incorporated a ultraviolet-B light source on the microscope. The glass used in standard microscope lenses blocks ultraviolet-B. Therefore, a 290–310 nm LED was introduced utilizing a light path that does not involve any of the microscope optics ( Fig. 4a ). In this setup, the cells were cultured on ultraviolet-B transparent poly-methyl-methacrylate (PMMA) coverslips, which were placed in quartz culture dishes. 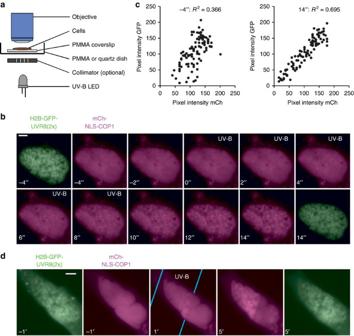Figure 4: Induction of H2B-GFP-UVR8(2x) and mCh-NLS-COP1C340interaction using an LED ultraviolet-B source. (a) Microscope setup. (b) Time-lapse images of U2OS cells expressing H2B-GFP-UVR8(2x) and mCh-NLS-COP1C340using the microscope setup shown in panel (a). The ultraviolet-B LED was turned on for 8 s (timepoints 0–8′′). Scale bar, 5 μm. (c) Linear regression analysis of the pixel intensities for the green (H2B-GFP-UVR8(2x)) and red (mCh-NLS-COP1C340) channels for the images acquired 4 s before ultraviolet-B illumination (left) and 14 s (right) after the start of ultraviolet-B illumination. The plots show only 100 randomly selected pixels for clarity. The correlation coefficients (R2) were calculated using the entire data set. (d) Ultraviolet-B-dependent interaction of H2B-GFP-UVR8(2x) and mCh-NLS-COP1C340in a subnuclear volume. Time-lapse images at the indicated times (in minutes) relative to the ultraviolet-B pulse are shown. The edges of the slit are indicated by the blue lines; the area between these lines was exposed to ultraviolet-B light. Scale bar, 5 μm. Figure 4: Induction of H2B-GFP-UVR8(2x) and mCh-NLS-COP1 C340 interaction using an LED ultraviolet-B source. ( a ) Microscope setup. ( b ) Time-lapse images of U2OS cells expressing H2B-GFP-UVR8(2x) and mCh-NLS-COP1 C340 using the microscope setup shown in panel ( a ). The ultraviolet-B LED was turned on for 8 s (timepoints 0–8′′). Scale bar, 5 μm. ( c ) Linear regression analysis of the pixel intensities for the green (H2B-GFP-UVR8(2x)) and red (mCh-NLS-COP1 C340 ) channels for the images acquired 4 s before ultraviolet-B illumination (left) and 14 s (right) after the start of ultraviolet-B illumination. The plots show only 100 randomly selected pixels for clarity. The correlation coefficients ( R 2 ) were calculated using the entire data set. ( d ) Ultraviolet-B-dependent interaction of H2B-GFP-UVR8(2x) and mCh-NLS-COP1 C340 in a subnuclear volume. Time-lapse images at the indicated times (in minutes) relative to the ultraviolet-B pulse are shown. The edges of the slit are indicated by the blue lines; the area between these lines was exposed to ultraviolet-B light. Scale bar, 5 μm. Full size image Using the setup described above, cells expressing H2B-GFP-UVR8(2x) and mCh-NLS-COP1 C340 were exposed to ultraviolet-B for 8 s, while being observed under the microscope. By the end of the 8 s period, the translocation of mCh-NLS-COP1 C340 from the nucleoplasm to chromatin had already reached a plateau ( Fig. 4b , Supplementary Movie 1 ). To quantify the COP1–UVR8 colocalization, we correlated the intensities of the pixels corresponding to the green (H2B-GFP-UVR8(2x)) and red channels (mCh-NLS-COP1 C340 ) over the entire nucleus of a cell before and after exposure to ultraviolet-B. Indeed, ultraviolet-B induced a considerable improvement in the R 2 linear regression coefficient ( Fig. 4c ). This improvement was also evident in two-dimensional plots of green and red channel intensities of 100 randomly selected pixels before and after ultraviolet-B illumination ( Fig. 4c ). To determine the minimal ultraviolet-B exposure time needed for the COP1–UVR8 interaction, we repeated the above experiment using subsecond exposure times. After a 0.4 s ultraviolet-B pulse, there was already partial colocalization of H2B-GFP-UVR8(2x) and mCh-NLS-COP1 C340 . The colocalization reached a plateau after an additional 0.4 s ultraviolet-B pulse ( Supplementary Movie 2 ). The ultraviolet-B LED setup described above allowed us to expose subcellular volumes to ultraviolet-B light. This was achieved by placing a collimator in the path of the ultraviolet-B light ( Fig. 4a ). The collimator that we used contains no optical lenses. It consists of silicon wafers that when stacked against each other form slits, whose width can vary between 1–10 μm. As the light path through the slits is several mm long, only rays of light that are parallel to the slits can pass through the collimator. We have previously described the use of this collimator for X-rays ( [14] , [15] ). Here we used a collimator with a light path length of 2.5 mm and a slit width of 10 μm placed about 1 mm away from the cells. Ultraviolet-B illumination of about half the nucleus of a cell expressing H2B-GFP-UVR8(2x) and mCh-NLS-COP1 C340 using this setup, resulted in chromatin recruitment of mCh-NLS-COP1 C340 only in the part of the nucleus that had been exposed to ultraviolet-B light ( Fig. 4d , Supplementary Movie 3 ). Thus, protein–protein interactions can be controlled spatially by controlling the pattern of ultraviolet-B illumination. γ−H2AX foci as indicators of ultraviolet-B-induced DNA damage One concern of using ultraviolet-B light to induce protein–protein interactions is the potential for ultraviolet-B-induced DNA damage. We therefore examined for the presence of γ−H2AX foci, which are markers of DNA damage [16] , in cells exposed to ultraviolet-B. When exposed to 25 J m −2 ultraviolet-B using the transilluminator, the cells showed considerable γ−H2AX signal, as expected ( Supplementary Fig. S7 ). In contrast, when illuminated with the ultraviolet-B LED for 0.5–1 s, an exposure sufficient for the UVR8–COP1 interaction to plateau, the γ−H2AX signal, although detectable, was weak ( Supplementary Fig. S7 ). The wavelength spectrum of ultraviolet-B emitted by the LED was quite narrow (290–310 nm) and within the range activating UVR8 ( [17] ). In contrast, the ultraviolet-B fluorescent lamps had an emission peak at 312 nm and a wide emission spectrum ranging from 280–370 nm. UVR8 responds poorly to wavelengths greater than 310 nm, yet these wavelengths can still induce DNA damage [17] , [18] , thereby explaining why the ultraviolet-B LED performed better than the ultraviolet-B fluorescent lamps present in the transilluminator. We have developed an optogenetic system to induce protein–protein interactions using the ultraviolet-B-dependent interaction between UVR8 and COP1. The system works efficiently in mammalian cells and does not require an exogenous chromophore. Further, the activation wavelength is such that the system does not interfere with imaging of the commonly used fluorescent proteins. On the negative side, the interaction between UVR8 and COP1, once induced, is essentially irreversible. Therefore, in its current form the system can be used to induce, but not disrupt, protein–protein interactions. However, in Arabidopsis we have recently demonstrated that the RUP1 and RUP2 proteins disrupt the interaction between UVR8 and COP1 ( [19] ), raising the possibility that in the future the optogenetic system described here may be adapted for reversible protein–protein interactions. In certain settings, the irreversible nature of the UVR8–COP1 interaction may be an advantage, as continuous exposure to ultraviolet-B light is not required to maintain the interaction. This is important, as prolonged exposure to ultraviolet-B light induces DNA damage. Indeed, using LEDs, instead of fluorescent tubes, as the ultraviolet-B source, and short pulses of illumination, we have been able to induce UVR8–COP1 interactions with minimal induction of DNA damage. In principle, the induction of DNA damage could be minimized even further, if the UVR8–COP1 interaction were induced by exposing only the cytoplasm to ultraviolet-B. Alternatively, two-photon lasers can excite Trps with 570–600 nm light. Thus, two-photon microscopy may allow high spatial resolution of UVR8 activation, while at the same time limiting ultraviolet-B induced damage. Finally, a unique property of UVR8 among the photoreceptors used so far in optogenetics is its mechanism of activation by monomerization of the UVR8 dimer. This unique mechanism could open up new strategies to control cellular processes by light. Plasmid construction The following primers were used (Sigma-Aldrich): Primer 1: AAAAAACCCGGGTATAGCAACGGCCTTGCAGATTTTCAATC Primer 2: AAAAGCGGCCGCTTACGCAGCGAGTACCAGAACTTTGATGG Primer 3: AAAGGATCCGCGGAGGATATGGCTGCCGACG Primer 4: AAAAGCGGCCGCTTAAATTCGTACACGCTTGACATCAGTTTG Primer 5: GTTTTATCTCCCAGATTTCGGGAGGTGCGAGACATACAATGGCATTGACTTCAG Primer 6: CTGAAGTCAATGCCATTGTATGTCTCGCACCTCCCGAAATCTGGGAGATAAAAC Primer 7: GTTTTATCTCCCAGATTTCGGGAGGTTTTAGACATACAATGGCATTGACTTCAG Primer 8: CTGAAGTCAATGCCATTGTATGTCTAAAACCTCCCGAAATCTGGGAGATAAAAC Primer 9: AAAAGCGGCCGCTTATCCGGAGTCTCCAGAGTCACCAATTCGTACACGCTTGACATCAGTTTGTGG Primer 10: AAAATCCGGAGATGGTTCTGGTGGTGACGGTTCTGGTGCGGAGGATATGGCTGCCGACG Primer 11: TTTTTCCGGAGCCTTTGCCACCCTTACCGTCTCCAGAGTCACCAATTCGTACACGC Primer 12: AATTCTAAGTGAGTAAAG Primer 13: GTCCTTTACTCACTTAG Primer 14: GTACGAATTGGTGACTCTGG Primer 15: AAAAGCGGCCGCTTATTACTTAAGACCAATTCGTACACGCTTGACATCAGTTTGTGG AccuPrime Pfx SuperMix (Invitrogen, 12344-040) was used for PCR-amplification. To generate the plasmid encoding mCh-NLS-COP1 C340 , COP1 C340 was amplified using primers 1 and 2, and inserted in a pSNV2-CHER-NLS vector with Xma I/ Not I. To generate the plasmid encoding GFP-UVR8, UVR8 was amplified using primers 3 and 4, and inserted in a pIRESN2-GFP vector with BamH I/ Not I. The UVR8 point mutations were introduced with primers 5 and 6 (W285A) and primers 7 and 8 (W285F), using the QuickChange Site-Directed Mutagenesis Kit (Stratagene). To generate the plasmid encoding H2B-GFP-UVR8, UVR8 was amplified using primers 3 and 4 and inserted in a pIRESN2-H2B-GFP vector with BamH I/ Not I. The plasmid encoding H2B-GFP-UVR8(2x) was generated in three steps. First a plasmid encoding H2B-GFP-UVR8 7aaLN was generated, which has a seven amino-acid long flexible linker. For this purpose, a region encoding part of the flexible linker flanked by a BspEI restriction site, a termination codon and a Not I site was introduced by amplifying UVR8 with primers 3 and 9, and insertion into the pIRESN2-H2B-GFP plasmid, using BamH I/ Not I. In the second step, a pIRESN2-H2B-GFP-UVR8 16aaLN -UVR8 plasmid was generated by amplifying UVR8 using primers 10 and 4, and insertion in the pIRESN2-H2B-GFP-UVR8 7aaLN plasmid, using Bsp EI/ Not I. Finally, the plasmid encoding H2B-GFP-UVR8 22aaLN -UVR8 or, in short, H2B-GFP-UVR8(2x), was generated by amplifying UVR8 16aaLN with primers 3 and 11 and insertion in the pIRESN2-H2B-GFP-UVR8 16aaLN -UVR8 plasmid, using Bam HI/ Bsp EI. The plasmid encoding GFP-UVR8(2x)-H3 was generated in three steps. First, a pIRESN2-GFP-UVR8(2x) plasmid was generated by deleting H2B from pIRESN2-H2B-GFP-UVR8(2x) using annealed primers 12 and 13 and Eco RI/ Ppu MI. Next, pIRESN2-GFP-UVR8(2x)-Afl2 was generated by amplifying pIRESN2-GFP-UVR8(2x) with primers 14 and 15 and inserting into the same vector using Bsp EI/ Not I. Finally, to generate pIRESN2-GFP-UVR8(2x)-H3, a histone H3 insert was cloned into pIRESN2-GFP-UVR8(2x)-Afl2, using Afl II/ Not I. For the mammalian transcription activation assays, UVR8 was amplified using primers 3 and 4 and inserted in the pCMV-AD vector (Stratagene) using Bam HI/ Not I to generate pCMV-AD-UVR8. COP1 C340 was amplified using primers 1 and 2, and inserted in pCMV-BD (Stratagene) using Bam HI/ Not I to generate plasmid pCMV-BD-COP1 C340 . Plasmids expressing firefly luciferase under the control of GAL4 (pFR-Luc) and Renilla luciferase under the control of a CMV promoter (pRL-CMV) were obtained from Stratagene and Promega, respectively. Cell culture and transfection U2OS cells (ATCC) were cultured in Dulbecco’s modified Eagle media (DMEM) (Gibco, 11960) supplemented with 10% FBS (Gibco, 10500) and 1 × penicillin-streptomycin-glutamine (Gibco, 10378). For transfection, cells were grown on 35 mm culture dishes (200,000 cells per dish) or on custom-made PMMA coverslips in wells of 12 well-plates (100,000 cells per well). The next day, 1 μg of each plasmid was added to a 100 μl volume of OPTI-MEM I (Gibco, 31985); FuGENE HD (Roche, 04709713001) transfection reagent was subsequently added (3 μl per μg DNA). After 25 min incubation at room temperature, this mixture was added to the cells. Two days later, the cells were analysed by fluorescence microscopy before and after exposure to ultraviolet-B. Ultraviolet-B treatment To activate UVR8, cells were exposed to ultraviolet-B using either ultraviolet-B fluorescent tubes or a ultraviolet-B LED. Ultraviolet-B fluorescent tubes The cells were irradiated by placing the dish, with the medium removed, in a CL-1000M Ultraviolet Crosslinker (UVP, 95-0230-02) equipped with five 8 W ultraviolet-B lamps (UVP, 34-0042-01) having a peak wavelength of 312 nm (emission spectrum range: 280–375 nm). Unless stated otherwise, the dose administered was 25 J m −2 . For the nuclear retention experiment, the cells were analysed by fluorescence microscopy at the indicated times after exposure to ultraviolet-B. For the chromatin recruitment experiment, the cells were analysed by fluorescence microscopy within seconds after exposure to ultraviolet-B. Ultraviolet-B LED The cells were grown on custom-made PMMA coverslips placed in quartz culture dishes (Labexchange). A UVTOP295 295 nm ultraviolet-B LED (SETI) set to operate at 20 mA with a typical power output of 0.7 mW and a peak wavelength of 300 nm (range 290–310 nm) was customized to fit in the condenser carrier of an upright microscope (Zeiss). Optionally, a commercially available collimator (2.5 mm light path; 10 μm slit width, MicroLeman) was placed between the ultraviolet-B LED and cells. Imaging Fluorescence images were acquired using a Zeiss AXIO Imager M.1 upright microscope, equipped with filter sets for DAPI, GFP and RFP (Chroma) and an X-Cite series 120 mercury vapour short arc light source (Lumen Dynamics). Images were captured with an ORCA-ER camera (Hamamatsu). Achroplan × 40/0.8 and Achroplan × 100/1.0 water immersion objectives were used for live cell imaging and an EC Plan-NEOFLUAR × 40/1.3 oil immersion objective was used for imaging of fixed cells. For data processing, the ImageJ (NIH) distribution FIJI was used. Images were enhanced by background subtraction, and linear adjustment of the image brightness and contrast. Statistical analysis To determine the nuclear fraction of GFP-UVR8 in cells co-expressing mCh-NLS-COP1 C340 before and after exposure to ultraviolet-B light ( Fig. 1d ), images of 25 cells per condition were acquired. Masks corresponding to the nucleus and plasma membrane of the cell were used to identify pixels corrresponding to the nuclear and total cellular volumes, respectively. The intensity values of these pixels were summed and used to calculate the fraction of nuclear GFP fluorescence for each cell. Means and s.d. of these fractions were then calculated. To determine the pattern (nucleoplasmic, partially nucleoplasmic or chromatin-bound, Fig. 2e ) of mCh-NLS-COP1 C340 localization in U2OS cells expressing mCh-NLS-COP1 C340 together with either H2B-GFP-UVR8(2x), H2B-GFP-UVR8 W285A (2x), H2B-GFP-UVR8 W285F (2x) or H2B-GFP, images of nuclei were acquired before and after exposure to ultraviolet-B. For each condition, five independent experiments were performed and from each experiment images of at least 20 nuclei were acquired. The five experiments were used to calculate means and s.e. of the fraction of nuclei exhibiting a specific mCh-NLS-COP1 C340 localization pattern. To quantify mCh-NLS-COP1 C340 and H2B-GFP-UVR8(2x) colocalization in U2OS cells ( Fig. 4c ), images acquired before (−4 s) and after (14 s) ultraviolet-B illumination were processed using ImageVision software (Silicon Graphics, Inc.). Briefly, a mask corresponding to the nucleus of a cell was used to select only the pixels corresponding to the nuclear area. The pixel intensity values from the red and green channels were used to calculate the R 2 correlation coefficient using linear regression analysis. The number of pixels used in the analysis was 101,016 for the images acquired before exposure to ultraviolet-B and 103,254 for the images acquired after exposure to ultraviolet-B. For a graphical representation, the intensity values of 100 randomly selected pixels were plotted. Two-hybrid transcription activation assays Mammalian cells A plasmid mix consisting of 1 μg pCMV-AD-UVR8, 1 μg pCMV-BD-COP1 C340 , 0.2 μg pCMV-RL and 0.5 μg pFR-Luc was transfected into U2OS cells grown in 3,5 mm dishes. To measure time dependency, similarly-treated plates of cells were exposed to a ultraviolet-B dose of 25 J m −2 using the transilluminator at 48, 49, 50, 51, 52 or 53 h after transfection. Luciferase activity was determined 1 h after the last exposure to ultraviolet-B. To measure dose dependency, 48 h after transfection, the cells were exposed to the indicated dose of ultraviolet-B and luciferase activity was determined 4 h later, using the Dual-Glo Luciferase Assay System (Promega). Yeast cells The yeast two-hybrid assay was performed, as previously described [7] . Ultraviolet-B induced γ−H2AX focus formation U2OS cells grown on PMMA coverslips were irradiated using the ultraviolet-B LED for 0, 0.5, 1, 3, 10 and 30 s, respectively, or exposed to 25 J m −2 ultraviolet-B using the ultraviolet-B transilluminator. Two hours after exposure to ultraviolet-B, the cells were fixed and processed for immunofluorescence using a rabbit histone H2AX Ser139 phosphospecific antibody (Cell Signaling, 2577, dilution 1:2,500) and secondary Alexa Fluor 594 goat anti-rabbit IgG (H+L) (Invitrogen, A11012, dilution 1:1,000). How to cite this article: Crefcoeur, RP. et al . Ultraviolet-B-mediated induction of protein–protein interactions in mammalian cells. Nat. Commun. 4:1779 doi: 10.1038/ncomms2800 (2013).